The function of fin rays as proprioceptive sensors in fish The sensation of movement and position of the limbs is critical for normal behaviours in tetrapods. In the bony fishes it is unclear what proprioceptive feedback is provided from the paired fins, the piscine homologues of the tetrapod limbs. Here we test mechanosensory abilities of afferent nerves in the pectoral fin rays, limb structures used by many fish species in propulsion and manoeuvreing. We examine the bluegill sunfish, a fish that uses its pectoral fins extensively in locomotion. We find that the activity of fin ray nerve fibres reflects the amplitude and velocity of fin ray bending. Spike sorting analyses demonstrate the presence of both slowly and rapidly adapting afferent nerve fibres. The fin sensory abilities we describe substantially expand the diversity of known vertebrate proprioceptive capabilities, and suggest that the pectoral fins need to be considered as possible proprioceptive sensors in studies of their functional morphology, movement and evolution. Unlike tetrapods, in which limb movement occurs at several discrete joints, the fins of ray-finned, actinopterygian, fishes include both proximal jointed elements and distal soft fin rays. The fin rays and the adjoining fin membrane are often highly flexible allowing for significant deformation during movement or in response to perturbation [1] , [2] . While many species of ray-finned fish use fin rays for propulsion and manoeuvreing [3] , [4] , [5] , fishes’ ability to sense fin ray movement during swimming is unknown. This is in contrast to sarcopterygian (including tetrapods) and chondrichthyan (sharks and their relatives) species that have a more extensive history of limb proprioception research [6] , [7] , [8] , [9] . However, electrophysiological recordings indicative of proprioceptive capabilities, from specialized filamentous pelvic fins in hakes [10] and from proximal joints of the three isolated pectoral fin rays of searobins [11] , suggest proprioception may be fundamental to fin movement in ray-finned fish species that are highly specialized for tactile foraging. Here we investigate proprioceptive sensation associated with the fin rays and membrane of the bluegill sunfish ( Lepomis macrochirus ), a species that uses its fins extensively for more typical movements, locomotor propulsion and manoeuvreing [12] , [13] , [14] . Neuroanatomy We found bluegill pectoral fins to be heavily innervated with fibres derived from four pectoral fin nerves. Collectively these nerves innervate the fin base, including fin musculature, and a subset of fibres extends distally to innervate individual fin rays ( Fig. 1a ). Each fin ray receives a nerve branch that enters the ray distal to its base and extends through the fin ray core formed by paired hemitrichia ( Fig. 1b ). The nerves within the fin rays are comprised of numerous fibres, some of which extend nearly the full length of the rays. These nerve fibre bundles divide to follow the branching pattern of the fin ray. Along the proximodistal length of the fin ray, nerve fibres diverge from the ray’s core to innervate the peripheral fin membrane ( Fig. 1c ). The general lack of muscle in or around the rays [2] and the lack of motor end plate-like structures [15] , [16] suggest that these nerves are, for the most part, sensory. While fishes are known to use fins for many forms of sensation [10] , [11] , [17] , the diversity of sensory endings and their functions has not been surveyed in detail, limiting interpretation of sensory capabilities from afferent morphology. 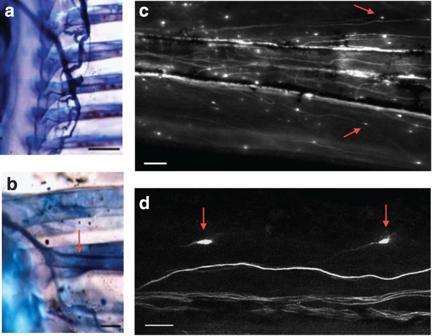Figure 1: Nerve staining in the pectoral fin rays. (a) Sudan black staining of pectoral fin nerves show nerves (black) tracking towards the fin rays and branching to enter the rays. Scale bar, 1 mm. (b) Nerve fibres enter the fin rays at their bases and extend through the core of the ray (arrow). Scale bar, 0.4 mm. (c) Anti-acetylated tubulin nerve staining shows that fibres follow the branching rays distally, as shown on the right side of the image. Nerve fiber endings are distributed through the fin membranes (arrows). Scale bar, 100 μm. (d) Expanded endings of afferents can be observed on many of the processes shown (arrows). Scale bar, 20 μm. Figure 1: Nerve staining in the pectoral fin rays. ( a ) Sudan black staining of pectoral fin nerves show nerves (black) tracking towards the fin rays and branching to enter the rays. Scale bar, 1 mm. ( b ) Nerve fibres enter the fin rays at their bases and extend through the core of the ray (arrow). Scale bar, 0.4 mm. ( c ) Anti-acetylated tubulin nerve staining shows that fibres follow the branching rays distally, as shown on the right side of the image. Nerve fiber endings are distributed through the fin membranes (arrows). Scale bar, 100 μm. ( d ) Expanded endings of afferents can be observed on many of the processes shown (arrows). Scale bar, 20 μm. Full size image Proprioceptive physiological responses We examined the physiological responses of fin ray afferents to movement and position of the fin rays ( Fig. 2 ). The nerve fibres recorded in the preparation did not branch to the muscles or tissues at the fin ray base. Fin rays responded to step-and-hold stimuli with bursts of increased spike rate (one-way analysis of variance (ANOVA), F =520.69, P <0.0001, 238 stimuli, seven individuals, comparing with baseline rates) at both the beginning and the end of the step. The duration of the burst of activity associated with initial deflection increased with increasing bend amplitude when assessed across all individuals and amplitude steps (one-way ANOVA, F =12.47, P <0.0001, 238 stimuli, seven individuals) ( Fig. 2b top). Overall the spike rate of the bursts also increased significantly (one-way ANOVA, F =5.91, P <0.0001, 238 stimuli, seven individuals). Owing to variability among individuals, regressions were performed independently on the data for each animal, shown in Fig. 2c (top), with regression equations are listed in Table 1 . For both duration and spike rate, a subset of fish did not demonstrate significant regressions. This variability among individuals is possibly due to the differences in the afferent fibre population recorded in each preparation. Overall, these data indicate that the bluegill pectoral fin rays have the ability to sense bending and suggest that the level of nerve activity observed reflects bend amplitude and may carry information about the extent of fin movement. 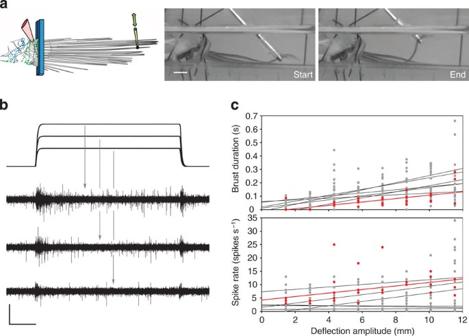Figure 2: Fin ray bending resulted in increased activity of the pectoral fin nerves. (a) Left panel: This illustration depicts the isolated fin electrophysiology preparation. Green lines represent nerve branches innervating in the fin rays, blue lines show nerve fibres innervating the pectoral fin muscles. The red cone represents the position of the extracellular recording electrode, just proximal to the afferent nerve’s exit from the fin rays. The nerves sampled in the preparation enter the rays distal to the joint of the rays with the proximal skeleton. No new nerve branches enter the nerve between the electrode and where the nerve enters the rays. A linear motor was used to actuate individual fin rays (yellow actuator attached to fin ray on right). Middle and right panels show the start and end of a fin ray deflection by an actuator in a step-and-hold stimulation trial. Scale bar, 5 mm. (b), Physiological responses to three bend amplitudes (top): 5.76 mm, 8.64 mm, and 11.52 mm. Scale bar,x=1s,y=0.04 mV. (c) Linear regressions show that, in a subset of individuals, increasing the amplitude of fin ray bending resulted in an increase in the duration of the corresponding burst of nerve activity (c, top) and at high amplitudes, increased activity when the fin ray was held in the bend position (c, bottom). Across all individuals both burst duration (one-way ANOVA,F=12.47,P<0.0001) and firing rate during the hold period increased with increasing step amplitude (one-way ANOVA,F=14.53,P<0.0002). Regression lines and data points in red are example data from a single fish. Data were collected from seven bluegill pectoral fins, with four to five repetitions of eight stimuli (238 stimuli). Figure 2: Fin ray bending resulted in increased activity of the pectoral fin nerves. ( a ) Left panel: This illustration depicts the isolated fin electrophysiology preparation. Green lines represent nerve branches innervating in the fin rays, blue lines show nerve fibres innervating the pectoral fin muscles. The red cone represents the position of the extracellular recording electrode, just proximal to the afferent nerve’s exit from the fin rays. The nerves sampled in the preparation enter the rays distal to the joint of the rays with the proximal skeleton. No new nerve branches enter the nerve between the electrode and where the nerve enters the rays. A linear motor was used to actuate individual fin rays (yellow actuator attached to fin ray on right). Middle and right panels show the start and end of a fin ray deflection by an actuator in a step-and-hold stimulation trial. Scale bar, 5 mm. ( b ), Physiological responses to three bend amplitudes (top): 5.76 mm, 8.64 mm, and 11.52 mm. Scale bar, x =1s, y =0.04 mV. ( c ) Linear regressions show that, in a subset of individuals, increasing the amplitude of fin ray bending resulted in an increase in the duration of the corresponding burst of nerve activity ( c , top) and at high amplitudes, increased activity when the fin ray was held in the bend position ( c , bottom). Across all individuals both burst duration (one-way ANOVA, F =12.47, P <0.0001) and firing rate during the hold period increased with increasing step amplitude (one-way ANOVA, F =14.53, P <0.0002). Regression lines and data points in red are example data from a single fish. Data were collected from seven bluegill pectoral fins, with four to five repetitions of eight stimuli (238 stimuli). Full size image Table 1 Regression equation variables. Full size table As limb proprioception includes sensation of both movement and static position, we examined the response of the fin ray to being held in fixed, deflected positions of various amplitudes by assessing activity during the hold interval of step-and-hold stimuli ( Fig. 2b ). Across stimulations, spike rates of a 3-s portion of the 5-s hold interval were compared with a 0.5 s prestimulus baseline. The 3-s portion of the hold period began 1 s after the step onset, to prevent inclusion of activity in response to the deflection. The spike rate for this period was significantly higher than for the 0.5-s prestimulus baseline ( F =8.39; one-way ANOVA, P =0.004, 238 stimuli, seven individuals). There were significant differences in spike rate among bend amplitudes with spike rate increase with increasing bend amplitude (one-way ANOVA, F =14.53, P <0.0002, 238 stimuli, seven individuals, Fig. 2c bottom). As can be seen in Table 1 and Fig. 2c (bottom), and similar to other kinematic parameters, regressions of some individuals have positive slopes while others do not. We suggest this is due to the types of afferents recorded and/or the position of the sensory ending along the proximodistal axis of the ray. The elevation in activity above baseline while the fin is held in a bent position and the difference in activity between deflection amplitudes in some individuals suggest that fin ray position—and not just bending movement—may be reflected in the nerve activity. To dissect further how nerve activity reflects movement of the fin rays, we applied ramp-and-hold and sinusoidal actuation protocols in our fictive fin preparation. We used ramp-and-hold stimulations to examine how the fin ray nerves responded to different displacement speeds. To separate effects of displacement distance from movement speed, we varied the ramp duration while holding the final amplitude of displacement constant and examined spike rate averaged across the duration of the ramp. We found that across the data set there was a gradual trend of increasing spike rate during the ramp portion of the stimulus corresponding to increasing ramp speed (one-way ANOVA, F =124.14, P <0.0001, 290 stimuli, seven individuals Fig. 3 ). Regressions of average activity rate during the bin against speed of deflection of the ray yielded R 2 -values over 0.5 and significance levels of P <0.0001 for all but one individual ( Table 1 ). This finding indicates that afferent firing rate is dependent on the rate of deflection above a threshold deflection speed of one centimeter per second. To determine whether the afferent activity observed could occur on time scales relevant to fin swimming, we used sinusoidal stimulation to actuate the fin rays within a normal range of fin beat frequencies, between 0.5 Hz and 3 Hz ( Fig. 4a ). The Hodge-Ajne statistical test [18] , [19] was performed for responses to each sinusoidal stimulus to determine whether the distributions of action potentials elicited by the cyclic stimuli were significantly non-uniform when summed across multiple cycles of stimulation, indicating periodicity in the afferent response. Across individuals, sinusoidal stimuli at 3 Hz were shown to regularly elicit periodic responses (83%), while response periodicity decreased overall with decreasing frequency. These results suggest that the velocity of fin ray displacement is among the proprioceptive cues available to the fish during movements of the pectoral fin and that afferent input can reflect typical oscillatory fin beat frequencies during swimming. 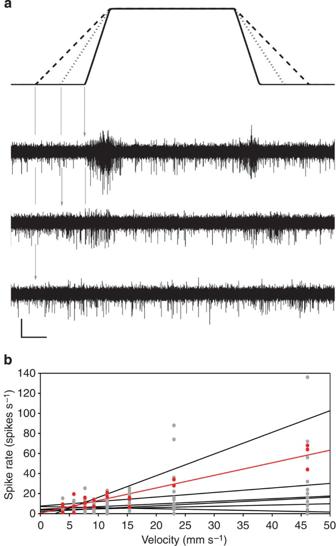Figure 3: Nerve activity reflected the speed of fin ray deflection in ramp-and-hold stimuli. (a) Increasing the ramp velocity to a set amplitude in the hold period resulted in increased pectoral fin nerve activity indicating that velocity as well as amplitude of fin ray bending is reflected in the afferent signal. Responses to 3.84, 5.76, and 11.52 mm s−1ramps are shown. Scale bar,x=1 s,y=0.03 mV. (b) Regression analyses show an increase in spike rate during the ramp portion of the stimulus corresponding with increasing ramp speed. This trend was found to be significant across the entire data set (one-way ANOVA,F=124.14,P<0.0001). The red regression line and data points are example data from a single fish. Data were collected from five fins with three to five repetitions of 12 stimuli (290 stimuli). Figure 3: Nerve activity reflected the speed of fin ray deflection in ramp-and-hold stimuli. ( a ) Increasing the ramp velocity to a set amplitude in the hold period resulted in increased pectoral fin nerve activity indicating that velocity as well as amplitude of fin ray bending is reflected in the afferent signal. Responses to 3.84, 5.76, and 11.52 mm s −1 ramps are shown. Scale bar, x =1 s, y =0.03 mV. ( b ) Regression analyses show an increase in spike rate during the ramp portion of the stimulus corresponding with increasing ramp speed. This trend was found to be significant across the entire data set (one-way ANOVA, F =124.14, P <0.0001). The red regression line and data points are example data from a single fish. Data were collected from five fins with three to five repetitions of 12 stimuli (290 stimuli). 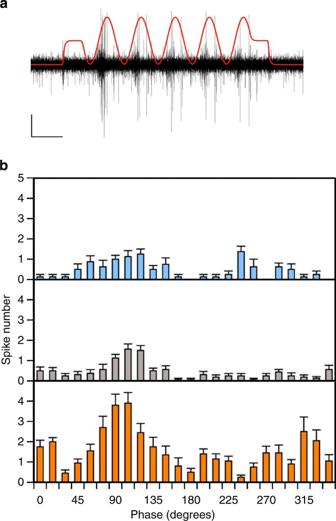Figure 4: Pectoral fin ray afferents respond cyclically to oscillations in the normal frequency range. (a) Multiunit response of pectoral fin ray nerve to a unilateral 1 Hz sinusoidal oscillation. (b) The number of action potentials observed during an oscillation showed a cyclic response that corresponded to the phase of the sinusoidal stimulation. Each panel shows responses of an individual to a 1-Hz sinusoidal stimulation. Spike counts were averaged in 15° bins over the course of a 360° oscillation cycle (top panel, eight trials; middle, 16 trials; bottom, 20 trials). Error bars represent the s.e.m. The cycle of the oscillation has been normalized so that 0°/360° corresponds to the resting position of the fin ray, and 180° corresponds to the point of maximum point of fin ray deflection during the sinusoidal bend. Full size image Figure 4: Pectoral fin ray afferents respond cyclically to oscillations in the normal frequency range. ( a ) Multiunit response of pectoral fin ray nerve to a unilateral 1 Hz sinusoidal oscillation. ( b ) The number of action potentials observed during an oscillation showed a cyclic response that corresponded to the phase of the sinusoidal stimulation. Each panel shows responses of an individual to a 1-Hz sinusoidal stimulation. Spike counts were averaged in 15° bins over the course of a 360° oscillation cycle (top panel, eight trials; middle, 16 trials; bottom, 20 trials). Error bars represent the s.e.m. The cycle of the oscillation has been normalized so that 0°/360° corresponds to the resting position of the fin ray, and 180° corresponds to the point of maximum point of fin ray deflection during the sinusoidal bend. Full size image Spike sorting Using spike sorting to interpret the unit responses that made up our multiunit recordings, we found that certain afferents only spiked during fin ray bending, while others continued firing through the hold interval ( Fig. 5 ). These data indicate that the populations of sensory neurons we recorded from are heterogeneous and include both slowly and rapidly adapting nerve fibres. Slowly adapting afferents ( Fig. 5 , top) displayed a distinctly increased firing rate in response to the hold intervals of the step-and-hold stimuli. Rapidly adapting afferents ( Fig. 5 , bottom) responded with a high firing rate during displacements, and were largely quiescent while the fin ray was statically bent during the hold periods of the stimuli. These data indicate that there are at least two fundamentally different proprioceptive afferents in the bluegill fin rays. 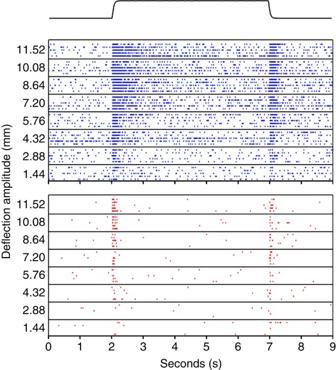Figure 5: Spike sorting of multiunit recordings. Spike rasters for a slowly adapting unit (top, blue) and rapidly adapting unit (bottom, red) show differing responses to step-and-hold stimuli. Each box contains five responses to a given stimulus amplitude arranged vertically. The onset and offset of the stimuli occur at 2 and 7 s, respectively. Five slowly adapting units and 28 rapidly adapting units were identified through spike sorting multiunit recordings collected from five bluegill. Figure 5: Spike sorting of multiunit recordings. Spike rasters for a slowly adapting unit (top, blue) and rapidly adapting unit (bottom, red) show differing responses to step-and-hold stimuli. Each box contains five responses to a given stimulus amplitude arranged vertically. The onset and offset of the stimuli occur at 2 and 7 s, respectively. Five slowly adapting units and 28 rapidly adapting units were identified through spike sorting multiunit recordings collected from five bluegill. Full size image Our findings, which indicate that pectoral fins not only serve as propulsors but also provide sensory feedback on fin mechanics, significantly change how we think about fin function in ray-finned fishes. The focus of previous mechanosensation research in teleost fins has been on fins thought to be specialized for tactile sensation [10] , [11] . Bluegills have a relatively typical pectoral fin morphology and possess similar innervation patterns to other ray-finned fishes [20] , [21] , [22] , suggesting that the fin proprioceptive sensation we recorded may be a widespread feature of teleosts. It is possible that such proprioceptive function provides feedback to tune motor output and/or that fins can function independently as sensors. Limb proprioception appears common to all three major extant vertebrate groups with limbs, including chondrichthyans, actinopterygians and sarcopterygians. This suggests that limb proprioception is a primitive feature for the gnathostomes (jawed vertebrates). Comparative studies of actinopterygians and sarcopterygians may provide insight into the evolution of both peripheral and central proprioceptive systems. Additionally, fin rays appear to be a primitive feature of sarcopterygian fins [23] . Investigating proprioceptive mechanisms in the fin rays of actinopterygian fishes may inform our understanding of how proprioception in tetrapod limbs arose. The presence of proprioception in the swimming fins of ray-finned fishes provides a new perspective on how this diverse group of vertebrates gathers information about its limb position and may have implications for a wide range of behaviours, including feeding, swimming and predator avoidance. Fin proprioception may also contribute to interactions within and between fish species. This proprioceptive sense could be a factor during interactions with potential mates and in caring for offspring, as well as, predator/prey interactions and in certain mutualistic contacts between fishes [24] . As in tetrapods, input from multiple sensory modalities is integrated to drive and modulate behaviours in fishes. This finding additionally raises questions of how the proprioceptive system interacts with other sensory systems such as the lateral line, the vestibular system and vision to generate an integrated picture of fin and body movement. Animals Adult bluegill ( Lepomis macrochirus ) were obtained from Keystone Hatcheries (Richmond, IL) and housed in aquaria at 20–23 °C with a standard seasonal light/dark cycle. Specimens ranged in size from 7.9 to 19.5 cm total length and 6.6 to 16.6 cm standard length. Fish used for physiological and morphological study (Sudan Black staining and immunocytology) were euthanized in a 0.5 g l −1 solution of MS-222 (Tricaine methanesulfonate, Sigma-Aldrich, St. Louis, MO) in water. The University of Chicago’s Institutional Animal Care and Use Committee approved all protocols for fish housing and euthanasia. Sudan black staining For Sudan Black staining, a modified protocol combining the methods of Song and Parenti [25] and Filipski and Wilson [26] was used. Fish were fixed in 10% formalin solution for ~1 week, followed by a 1-week rinse in deionized water. The fins were removed and placed in a trypsin solution until muscles became translucent. Specimens were gradually dehydrated to 70% ethanol and placed in a 30% Sudan Black B (Sigma-Aldrich) solution overnight. After rehydrating, the fins were placed back in trypsin until nerves were clearly visible. All specimens were then soaked in 0.5% KOH solution overnight and gradually stepped up to 100% glycerol for storage. Six fins from four individuals were used for staining overall pectoral girdle innervation. Five fins from three individuals were stained to examine the innervation at the base of the fin rays. Antibody staining Immunocytology was used to label nerves innervating the pectoral fin rays and fin membrane of seven adult bluegills. Methods for immunocytology follow those found in Thorsen and Hale [22] . For six of the seven specimens, a monoclonal antibody to a neurofilament-associated protein (3A10, Developmental Studies Hybridoma Bank, Iowa City, IA) was used as the primary antibody. Mouse monoclonal anti-acetylated tubulin (Sigma-Aldrich) was used as the primary antibody in the seventh specimen. The secondary antibody used in the labelling of the fin nerves was a goat antimouse antibody conjugated with fluorescein (five specimen, Jackson ImmunoResearch Laboratories, West Grove, PA) or rhodamine (two specimen, Jackson ImmunoResearch Laboratories). Primary and secondary antibodies were applied at a 1:100 ratio of antibody to solution of bovine serum albumin, phosphate buffered saline and Tween-20. Fluorescent images of the labelled nerve fibres were collected with an inverted microscope and laser-scanning confocal imaging system (Zeiss LSM 510, Thornwood, NY). Stimuli Fin ray bending stimuli in the physiological experiments were performed using an actuator mounted on a voice coil positioning stage (VCS10-023-BS-01-M, H2W Technologies Inc., Valencia, CA) that was controlled by a programmable driver (Intelligent Servo Drive IDM640-8EI, Technosoft, Canton, MI). The Somlab software system (developed by John F. Dammann III, University of Chicago) was used to generate stimuli to programme the driver. Randomly presented series of step-and-hold stimuli (1.44, 2.88, 4.32, 5.76, 7.20, 8.64, 10.08 and 11.52 mm), and ramp-and-hold stimuli (3.84, 4.19, 4.608, 5.12, 5.76, 6.58, 7.68 9.22, 11.52, 15.36, 23.04 and 46.08 mm s −1 ), were used to examine responses during fin bending. All ramp-and-hold stimuli were deflected to an amplitude of 11.52 mm. All step-and-hold and ramp-and-hold had 5-s hold intervals. Low frequency sinusoidal stimuli (0.5, 1, 1.5, 2, 2.5 and 3 Hz) were also used, presented in randomized order. These frequencies were designed to examine responses to fin ray bending frequencies similar the fin beat cycle of the bluegill during the low speed swimming. All stimulation trials were filmed with a Fastcam APX RS camera (Photron, San Diego, CA), at 125 fps, to compare properties of fin ray bending with the recorded physiological responses. Electrophysiology We used extracellular recordings to examine the electrophysiological response of pectoral fin nerve fibres to fin ray bending. Eleven adult bluegill were used in these sensory physiology experiments. Seven fish were used in step-and-hold experiments (238 stimuli). Seven individuals were used in ramp-and-hold experiments (290 stimuli). Three blugill were used in sinusoidal experiments (144 stimuli). Numbers of trials, broken down by individual and experiment, are provided in Table 1 . After the fish was euthanized, we removed the head of the animal to better access the pectoral fins. We then excised a pectoral fin of the bluegill along with a portion of the pectoral girdle. We removed the dermal layers covering the nerves innervating the fin rays, and pinned the fin through muscle and connective tissue to a petri dish with a Sylgard (Dow Corning, Midland, MI)-coated floor. The fin rays were clamped firmly near their proximal ends to limit movement beyond the rays. We cut through the fin membrane to isolate individual rays for bending. The preparation was bathed in extracellular solution, made according to the methods found in Masino and Fetcho [27] . Regularly through experiments, fresh extracellular solution was exchanged into the bath. We recorded multiunit physiological responses from nerves on the medial side of the fin innervating the fin rays using glass suction electrodes. Borosilicate glass capillaries (GC150F-7.5 1.5 mm OD, 0.86 mm ID, Harvard Apparatus, Holliston, MA), were pulled using a Flaming/Brown micropipette puller, model P-97 (Sutter Instrument Co., Novato, CA), and fire-polished with a microforge (MF-830, Narishige, East Meadow, NY) to create the electrodes. We used electrodes fashioned with tips ranging from 35–50 μm in diameter in our experiments, selecting electrodes with widths that corresponded best to the diameter of the pectoral fin nerves of the specimen. The electrodes were filled with extracellular solution and mounted on an Axon Instruments CV-7B headstage (Molecular Devices, Foster City, CA). The recording electrode was positioned along exposed portions of nerve at the base of the pectoral fin rays as they entered the rays and fin membrane, to obtain multiunit extracellular responses to fin ray bending stimuli. A MultiClamp 700B amplifier (Molecular Devices, Foster City, CA) in current-clamp mode to was used to monitor extracellular voltage. The voltage recordings were digitized with a DigiData 1440A digitizing board (Molecular Devices, Foster City, CA) and acquired using pClamp 10 software (Molecular Devices, Foster City, CA). Data analysis Physiological data, sampled at 100 kHz and down-sampled to 10 kHz, were filtered with a second-order elliptical filter and analyzed with MATLAB 7.10.0 (Mathworks, Natick, MA). To eliminate transient effects associated with the initialization of mechanical stimulation, the first stimulus of each step-and-hold, and ramp-and-hold series was excluded from subsequent analyses. Similarly, the first cycle of sinusoidal stimuli were also excluded. Analysis of spike rate during the hold interval of step-and-hold stimuli was limited to a 3-s portion of the 5-s hold interval. The 3-s portion of the hold period began 1 s after the step onset, to prevent inclusion of activity in response to the deflection. This portion of the hold interval was compared to a 0.5 s prestimulus baseline. Analysis of variance was performed on the full data sets and ordinary least squares regressions were fit to each individual independently, due to differences in trial sample size and scaling. Statistical analyses of step-and-hold and ramp-and-hold stimulation data were performed with JMP software (SAS, Cary, NC). The MATLAB circular statistics toolbox, CircStat, was used to perform Hodges-Ajne tests on sinusoidal stimulation data [28] . We used a modified version of the Wave clus [29] spike sorting software, to detect, and sort action potentials in our recordings. Wave clus provides an unsupervised method of spike sorting using a super-paramagnetic clustering of spikes based on the wavelet features extracted from a four-level, multiresolution, Haar wavelet transform of each action potential. All firing rates were calculated as the number of action potentials observed divided by the duration of the observation time in seconds. A burst of action potentials was defined as three or more spikes occurring within 50 ms of each other. The first action potential recorded after the start of the onset of the stimulus was considered the beginning of a burst at the onset of the stimulus. The first action potential recorded after downward motion began after the hold period of the stimulus was considered the beginning of a burst at the offset of the stimulus. We classified individual spike sorted units as either rapidly or slowly adapting utilizing modified methods from Lichtenstein et al . [30] In the spike sorting analysis the firing rate of the unit during the initial 2 s of the hold interval of step-and-hold stimuli was compared with the firing rate observed during a 2-s prestimulus interval using two-tailed t -tests. Those units with a firing significantly greater during the hold interval ( P <0.025), as compared with the prestimulus interval, were classified as slowly adapting. Units that did not respond with a significantly greater firing rate were classified as rapidly adapting. How to cite this article: Williams IV, R. et al . The function of fin rays as proprioceptive sensors in fish. Nat. Commun. 4:1729 doi: 10.1038/ncomms2751 (2013).